EPR-aided approach for solution structure determination of large RNAs or protein–RNA complexes High-resolution structural information on RNA and its functionally important complexes with proteins is dramatically underrepresented compared with proteins but is urgently needed for understanding cellular processes at the molecular and atomic level. Here we present an EPR-based protocol to help solving large RNA and protein–RNA complex structures in solution by providing long-range distance constraints between rigid fragments. Using enzymatic ligation of smaller RNA fragments, large doubly spin-labelled RNAs can be obtained permitting the acquisition of long distance distributions (>80 Å) within a large protein–RNA complex. Using a simple and fast calculation in torsion angle space of the spin-label distributions with the program CYANA, we can derive simple distance constraints between the spin labels and use them together with short-range distance restraints derived from NMR to determine the structure of a 70 kDa protein–RNA complex composed of three subcomplexes. RNA is a crucial regulator of gene expression and its importance is exemplified by the fact that more than 98% of the transcribed DNA in humans does not code for proteins [1] . While structural information on RNA and its functionally important complexes with proteins is urgently required for understanding cellular processes at the molecular and atomic level, high-resolution structural information of RNAs and protein–RNA complexes are profoundly underrepresented compared with protein structures. RNA or its macromolecular complexes have inherent structural flexibility and might be present in multiple conformations that complicate crystallization [2] , [3] , [4] , [5] . Furthermore, crystallization presents the risk of trapping a single conformation out of multiple possible ones present in solution and of crystallization artefacts such as non-native macromolecular complex topologies and stoichiometries due to crystal packing effects [6] , [7] . Therefore, potentially dynamic RNA molecules or macromolecular complexes should preferentially be studied in solution. Efficient approaches for solution structure determination of large proteins and protein–protein complexes have successfully been applied by combining traditional NMR spectroscopy with the measurement of paramagnetic relaxation enhancement (PRE), residual dipolar coupling (RDC) data or with other biophysical methods such as small-angle X-ray scattering (SAXS) [7] , [8] , [9] , [10] , [11] . However, these approaches fail on large RNAs and their complexes due to high-resonance overlap, line broadening and low proton density found in the RNA part of such complexes [12] . This in turn reduces the number of high-quality RDC or PRE data that can be measured. Furthermore, macromolecules present in more than one conformation in solution considerably complicate the interpretation and analysis of RDC, PRE and SAXS measurements. In contrast, distances in a macromolecular complex can be measured under solution conditions by electron paramagnetic resonance (EPR) spectroscopy in a range that matches typical dimensions of such complexes with a resolution that is independent of the size of the complex [13] . Thus, valuable long-range distance distribution constraints could be obtained if pairs of site-specific spin labels were introduced. However, obtaining such distance constraints is limited by the difficulty for labelling such RNAs and the precision of the distances is dependent on the conformational distribution of the labels [14] . Here we introduce a new approach for the structure determination of large RNAs and protein–RNA complexes by combining a large number of short-range nuclear Overhauser effect (NOE) NMR restraints with a moderate number of long-range EPR distance constraints. This approach is used to investigate the structure of a 70-kDa protein–RNA complex consisting of the 72 nucleotides (nts) non-coding RNA RsmZ bound to three RsmE protein homodimers [15] , a complex regulating translation initiation in bacteria [15] , [16] ( Fig. 1a ). 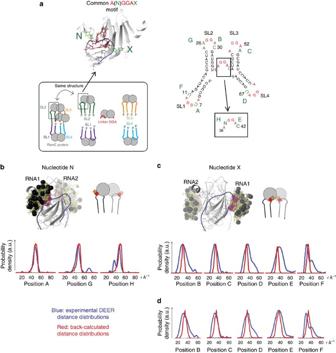Figure 1: Measuring and modelling distance distributions using a model system of two singly spin-labelled RNAs bound to RsmE. (a) The RsmZ(1–72)/RsmE 1:3 complex is composed of several domains, which have the same structure in isolation and in the full complex15. The common A(N)GGAX motif containing the unspecifically recognized nucleotides N and X is present at every protein-binding site. (b–d) The modelled distance distributions (red curves) for the common positions N (b) and X (c,d) are obtained by plotting all possible distances between the radical positions (black sphere) of RNA1 and RNA2. Experimental DEER data: blue curve. The experimental and simulated distance distributions were scaled to similar maximum amplitude. (d) Taking into account the flexibility of nucleotide X. By increasing the NOE upper limit restraints of the nucleotide X to the protein by 2 Å, the experimental and back-calculated distance distributions are in better agreement. Figure 1: Measuring and modelling distance distributions using a model system of two singly spin-labelled RNAs bound to RsmE. ( a ) The RsmZ(1–72)/RsmE 1:3 complex is composed of several domains, which have the same structure in isolation and in the full complex [15] . The common A(N)GGAX motif containing the unspecifically recognized nucleotides N and X is present at every protein-binding site. ( b – d ) The modelled distance distributions (red curves) for the common positions N ( b ) and X ( c , d ) are obtained by plotting all possible distances between the radical positions (black sphere) of RNA1 and RNA2. Experimental DEER data: blue curve. The experimental and simulated distance distributions were scaled to similar maximum amplitude. ( d ) Taking into account the flexibility of nucleotide X. By increasing the NOE upper limit restraints of the nucleotide X to the protein by 2 Å, the experimental and back-calculated distance distributions are in better agreement. Full size image Modelling spin-label distributions For small RNAs (less than 30–50 nts), site-specific introduction of spin labels is typically achieved by chemical synthesis of RNAs containing modified nucleotides to which spin labels are subsequently attached [17] . A commonly used and experimentally simple way to introduce spin labels into structured RNA without significantly altering the double-stranded RNA structure [18] is the attachment of the flexible 3-(2-iodoacetamido)-proxyl (IA-proxyl) spin label to a 4-thiouridine residue [19] . Using the IA-proxyl spin label, we first tested if we can measure and also successfully back-calculate known long-range distance distributions within a model protein–RNA complex system. All protein-binding sites in the RsmZ RNA consist of a common A(N)GGAX motif, in which the nucleotides N and X are non-sequence-specifically recognized by the RsmE protein, and thus can be replaced by a thiouridine residue to which a nitroxide spin label can be attached ( Fig. 1a ). By forming complexes between the homodimeric RsmE protein and two copies of each isolated RNA-binding site containing a spin label, complexes with two spin labels are obtained for which the structures without attached spin labels were recently determined using NMR at high precision [20] ( Fig. 1a ). We could then measure the distance distributions of several spin labels attached at different sites representing either of the two nucleotides N or X in the various binding sites ( Fig. 1b,c and Supplementary Fig. 1 ) and compare them with predicted distances after torsion angle dynamics simulations ( Fig. 1b–d ). Several approaches exist for modelling distance distributions between two spin labels. Long (4 ns) molecular dynamics simulations [21] and rotamer library approaches [22] have similar accuracy [14] . While rotamer library approaches are computationally faster, they require pre-calculated sets of nitroxide label conformations, which are currently available only for a very limited number of spin-label types. Simpler conformer search algorithms can also map the conformational space of nitroxide labels sufficiently well, but are so far restricted to the R5 nitroxide probe attached to a phosphorothioate in DNA or RNA [21] , [22] , [23] , [24] . Here we computed nitroxide label conformers with the well-established torsion angle dynamics simulations program CYANA [25] , which allows a straightforward application to a broad range of spin-label types. Including into the structure calculation all NOE NMR restraints from each protein–RNA complex, along with the 4-thiouridine to which the tag is attached and not constraining the spin label, allowed a simple and fast sampling of the spin-label conformations at every spin-label attachment site (see Methods section). After calculating 5,000 structures and superimposing the 50 with the lowest energy, we could compute with the structure ensemble a distance distribution by measuring all 2,500 (50 × 50) possible distances between the two radicals attached on the two RNA molecules bound to the protein. The mean distances of the experimental and computed distributions are in remarkable agreement ( Supplementary Table 1 ), which further indicates that the spin label does not affect the structure of the protein–RNA complex despite different solution conditions for EPR and NMR (EPR measurements are performed in 50% glycerol). For the sites corresponding to nucleotide N, the width of the distance distribution can also be reproduced well by the calculation ( Fig. 1b and Supplementary Table 1 ). In contrast, for the sites corresponding to nucleotide X, the width of the experimental distance distribution is broader than the modelled one ( Fig. 1c and Supplementary Table 1 ), indicating that these nucleotides are not entirely rigid, especially for position E that is in a single-stranded RNA. Indeed, we find a narrower line width of the 1 H– 13 C NMR resonances for the H5 and H6 protons of the X nucleotides, which is consistent with a partially mobile nucleotide. Subsequent simulations, in which the interNOE-derived distance restraints of the nucleotide X to the protein were increased by 2 Å to mimic increased flexibility, resulted in a better agreement between the width of measured and the modelled distance distributions ( Fig. 1d and Supplementary Table 1 ). Remarkably, the structures of RsmE bound to various RNA stem-loops [20] , [26] explain why the base of nucleotide X experiences more dynamics than the one of nucleotide N. While nucleotide N is well positioned with its base always sandwiched between the RsmE protein side chains of I47 and P58, this is not the case for the base of nucleotide X that packs against the protein side chains of M1 and L23, however, only on one side of the base [20] . Overall, the agreement between the experimental and computed results indicates that spin labels attached to the sites N and X of the different binding sites of RsmZ do not disturb the structure of the complex, and can therefore be reliably used to report on the precise distance between those sites, and that the conformer search with CYANA is a simple and efficient approach to model spin-label distributions even for partially dynamic nucleotides. Production of large spin-labelled RNAs Next, our aim was to measure such long-range EPR distances within the complete 70-kDa RsmZ–RsmE 1:3 complex. The large size of most biologically relevant RNAs prevents to obtain doubly spin-labelled RNAs simply by chemical synthesis. However, modified and unmodified RNA fragments can be ligated using enzymatic ligation [27] , [28] , [29] , [30] . To our knowledge, ligation to obtain large RNAs containing two nitroxide spin labels has not been reported yet, with the recent exception of a deoxyribozyme-catalysed ligation, which is limited by strict sequence requirements at the sites of ligation [31] . We investigated two possible strategies using splinted T4 DNA ligation. In the first approach, ligation of the 4-thiouridine-modified and -unmodified fragments is followed by spin labelling ( Fig. 2a ). In the second approach, the spin label is first attached to the 4-thiouridine-modified fragments, which are subsequently ligated with the unmodified RNA fragments ( Fig. 2b ). Following ligation, in both approaches the RNA of interest has to be separated from the different unreacted RNA fragments, the ligation RNA side products and the long DNA splint. Efficient separation of the different oligonucleotides with the highest possible yield requires a denaturing purification step at high temperature (85 °C) on an anion-exchange HPLC [28] . Following ligation of the unmodified and 4-thiouridine-containing fragments and subsequent purification by HPLC, the spin label could not be attached anymore, probably due to hydrolysis of the 4-thiocarbonyl groups. By first attaching the spin label and subsequently ligating the fragments (typical yields of 20–40%), spin-labelling efficiencies of 85–100% were obtained after purification for most doubly spin-labelled RNAs ( Fig. 2b ). With typical amounts required for double electron-electron resonance (DEER) EPR measurements (around 3 nmol for 30 μl of 100 μM spin-labelled RNA), <20 nmol of 4-thiouridine-modified RNA is required as starting material. 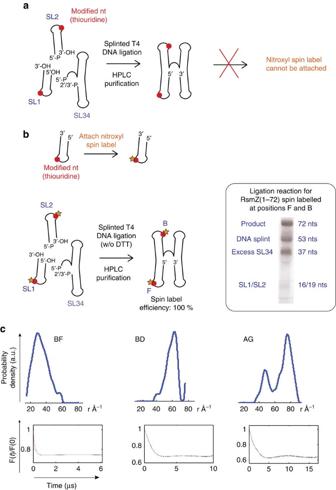Figure 2: Strategy for production of nitroxide spin-labelled RNAs and measurement of distances above 80 Å using DEER EPR spectroscopy. (a,b) Ligation performed before (a) or after (b) spin labelling. (c) DEER spectroscopic data measured on the RsmZ(1–72)/RsmE dimer 1:3 complex for RNAs labelled at different positions; distance distributions (top) and form factor DEER time traces (bottom). Figure 2: Strategy for production of nitroxide spin-labelled RNAs and measurement of distances above 80 Å using DEER EPR spectroscopy. ( a , b ) Ligation performed before ( a ) or after ( b ) spin labelling. ( c ) DEER spectroscopic data measured on the RsmZ(1–72)/RsmE dimer 1:3 complex for RNAs labelled at different positions; distance distributions (top) and form factor DEER time traces (bottom). Full size image We then formed the complexes of spin-labelled RsmZ(1–72) RNAs with three equivalents of deuterated RsmE protein dimer and verified the successful 1:3 complex formation by native polyacrylamide gels. Using 4-pulse DEER EPR spectroscopy, we were able to measure distances reliably above 80 Å, supported by the measurement of some long 16–18 μs primary DEER traces ( Fig. 2c and Supplementary Fig. 2 ). Importantly, our approach takes advantage of extensive sample deuteration [32] and high-power Q-band EPR [33] , which provides high signal-to-noise ratio at long observation times and thus access to long spin–spin distances. Overall, our procedure allows obtaining spin-labelled RNAs at any desired pair of sites and should permit to access RNAs of several hundred nucleotides. Thus, many biologically relevant RNAs and their complexes could become accessible for DEER measurements for measuring distances of up to 100 Å in a simple and efficient way. Protocol for structure determination After attaching the spin labels at two specific sites ( Fig. 3 , step 1) and measuring the distance distributions ( Fig. 3 , step 2), the experimental distributions have to be converted into simple constraints for structure calculation. To make the data fitting procedure fast and stable, it is better to use single constraints rather than complicated distribution analysis and fitting. In previous approaches, measured EPR DEER data were directly translated to distance constraints between Cα positions [34] or Cβ positions [35] of the labelling sites or assigned to the distance between the O atoms of an explicitly modelled nitroxide spin label [36] . Because the spin label is flexible, the radical position with respect to the backbone is not known a priori so that all these approaches are fraught with additional uncertainty. Mean distances are not much affected by the ill-posedness of the data conversion from time to distance domain [13] and there is a strong correlation between the experimental and CYANA-computed mean distances even for broad distance distributions ( Fig. 1 and Supplementary Table 1 ) [37] , [38] , [39] . The CYANA-computed mean distance corresponds in a good approximation to the distance between the geometrical centres of the two spin-label distributions (radical clouds) (see Supplementary Table 1 ). Therefore, we could derive simple EPR distance constraints by restraining the centres of the two radical clouds with the experimental mean distance. Because of the modular architecture of large RNAs or protein–RNA complexes, we first calculated the radical clouds on the isolated domains ( Fig. 1 ) and then superimposed those radical clouds onto the corresponding sites of the full RNA or protein–RNA complex ( Fig. 3 , step 3). For structure calculation with CYANA, we then placed a dummy atom at the geometric centre of each simulated radical cloud ( Supplementary Information ) and each dummy atom pair was restrained using lower and upper limits that confine a 70% probability around the maximum of the DEER distance distribution ( Fig. 3 , step 4). These broad distance ranges account for uncertainties in DEER data analysis and in simulations of the spin-label distributions. We folded the whole complex from random coil conformations using CYANA by including the local restraints, which determine the structure of the isolated domains (NOEs, dihedral angles, hydrogen bond restraints; Fig. 1a ), and the long-range EPR constraints ( Fig. 3 , step 5). Measuring a total of 21 long-range distances, we could calculate the 70 kDa structure of the 72 nts RsmZ(1–72) RNA bound to three homodimeric RsmE proteins (see ref. 15 for a detailed description of the structure and its functional implications). We could even resolve two conformations simultaneously present in solution. The superposition of some representative experimental DEER distance distributions with the back-calculated distributions using the final structural ensemble illustrates the internal consistency of our approach ( Fig. 3 , step 6). For further validating our structures, we did a cross-validation analysis by performing structure calculations in which a single distance constraint was omitted. For most structure calculations, we obtained comparable solutions indicating that the system is overdetermined and stable (see Methods). 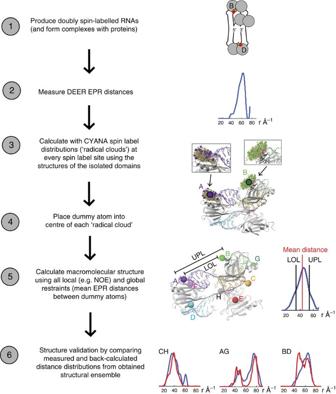Figure 3: General protocol for structure determination of large RNAs or protein–RNA complexes using EPR-derived distance constraints. . Figure 3: General protocol for structure determination of large RNAs or protein–RNA complexes using EPR-derived distance constraints. . Full size image Here we have described an approach for solution structure determination of large RNAs or protein–RNA complexes that takes advantage of a limited number of long-range EPR constraints to position several rigid domains with respect to each other. As EPR spectroscopy can measure distances independently of the size of a macromolecule and RNA and protein NMR resonances can be observed in high molecular weight complexes with appropriate isotope labelling schemes [27] , [30] , [40] , [41] , [42] , we expect this structural approach to be applicable to significantly larger RNAs or protein–RNA complexes than the 70 kDa RsmE–RsmZ complex described above. Also low affinity complexes (intermediate μM to low mM range) should be accessible by this methodology. Another salient feature of our approach is the possibility of determining more than one conformation simultaneously present in solution [15] , which is urgently needed since many larger RNAs and their complexes with proteins are dynamic in nature [2] , [3] . Although the measurement of EPR data requires the preparation of a separate spin-labelled sample for each distance to be measured, it has several advantages compared with other methods. Obtaining PRE or RDC data requires the acquisition of a large number of well-resolved resonance pairs of high quality. While this can be achieved for protein resonance pairs, it is significantly more difficult to obtain enough data of sufficient quality on the RNA part. First, the NMR resonances are clearly more overlapped in RNA than in proteins. Although segmental labelling of RNA can dramatically help to resolve such spectral overlap [27] , [28] , the production of many RNA samples is very time consuming and costly. Second, the proton density in RNA is smaller compared with that in proteins, reducing the number of observable resonances. Third, due to the fast relaxation of the sugar protons and the pyrimidine H5 and H6 protons, measurement of one-bond couplings is limited to purine H8, adenine H2 and the imino protons of the uracil and guanine in large RNAs or protein–RNA complexes, which further reduces the number of measurable RDCs or PREs on the RNA part [12] . This low density of observable RNA NMR resonances is especially critical for the measurement of PREs because they provide only medium-range distance information (20–25 Å). In contrast, EPR allows the measurement of long-range distances that typically correspond to the dimensions between different domains in large RNAs or protein–RNA complexes. The measurement of SAXS data has proved to be very valuable to obtain information on the global shape of macromolecules and their complexes [8] , [11] , [43] . However, SAXS data only provides low resolution information and has to be supplemented with data obtained by complementary biophysical methods such as PREs or RDCs. Furthermore, the interpretation of SAXS data can be difficult if the shape of the complex is more globular than extended, which is the case for the RsmE–RsmZ protein–RNA complex that was studied here. Finally, the presence of more than one conformation will clearly complicate the interpretation of the SAXS data and unlikely result in a successful structure determination. The new structure determination approach described here could be successfully implemented since the complex is composed of three rigid structures (three RsmE dimers bound to RNA) separated by short RNA linkers. The same approach is likely to be applicable for determining the structure of a multi-domain RNA-binding protein bound to RNA or the structure of an assembly of small RNA-binding proteins bound to RNA. However, it might not be directly applicable for determining the structures of large globular proteins bound to RNA. On large protein–RNA complexes composed of different protein domains and of proteins not being homodimeric, EPR distance constraints could also be obtained for the protein. In such systems, the EPR constraints could be supplemented by additional NMR-based restraints, such as RDC or PRE data or data from other biophysical methods like SAXS [7] , [8] , [9] , [11] . This would reduce the number of EPR distances to be measured to obtain a unique solution of high precision. In summary, we have presented a method to obtain large doubly spin-labelled RNAs, enabling the measurement of EPR distances above 80 Å in a large protein–RNA complex. The well-established NMR structure calculation program CYANA was used to model spin-label distributions in a simple way with good accuracy, providing a means for using EPR distance distributions as simple constraints for structure calculation. Taken together, this results in an efficient EPR-based procedure for solution structure determination of large RNAs or protein–RNA complexes that are not easily accessible by other techniques. RsmE protein expression and purification The RsmE protein from Pseudomonas fluorescens CHA0 was cloned into a pET28a vector with a C-terminal histidine tag. The hexahistidine-tagged RsmE protein was overexpressed in Escherichia coli BL21(DE3)+RIL at 37 °C in minimal M9 medium containing 1 g l −1 15 NH 4 Cl and 4 g l −1 unlabelled glucose (for 15 N-labelled proteins). The cell cultures were induced at OD600=0.6 with 1 mM isopropyl β-D-thiogalactoside for 4 h at 37 °C. After lysis of the cells, the supernatant was purified with Ni-NTA (nitrilotriacetic acid) metal-affinity chromatography. The fractions containing the pure protein were pooled and dialysed against NMR buffer (30 mM NaCl, 50 mM potassium phosphate at pH 7.2) and concentrated to ~1 mM. Aliquots (100 nmol) were frozen at −20 °C. Deuterated RsmE was obtained by growing the cells in ~90–99% D 2 O rather than H 2 O but using protonated glucose as carbon source. Preparation of doubly spin-labelled RsmZ RNAs Attachment of IA-proxyl spin label to modified RNA containing a 4-thiouridine Small RNAs (10–25 nts) containing a single 4-thiouridine modification at a specific position were purchased from Dharmacon and deprotected according the manufacturer’s instructions. The IA-proxyl spin label was attached to the modified RNA according to an adapted protocol from Ramos and Varani [19] . The IA-proxyl spin label was dissolved in 100% methanol to obtain a 100 mM concentration. The modified RNA was resuspended into reaction buffer containing 100 mM potassium phosphate at pH 8.0, 80–110 μM 4-thiouridine-modified RNA and 8–11 mM IA-proxyl spin label (100-fold molar excess over modified RNA). The reaction mix was incubated for 20–28 h at 25 °C in the dark under vigorous shaking. The spin-labelled RNA was purified using a buffer exchange NAP-10 column from GE healthcare. All the fractions having an absorption ratio A260/230 of >1 were collected. The RNA concentration was determined by UV spectroscopy. If the RNA was directly used for EPR measurements without further ligation (for the complexes shown in Fig. 1 ), the purified RNA was subjected to a second NAP-10 column purification step. RNase H cleavage and ligation To obtain the full-length doubly spin-labelled RNAs, two singly spin-labelled RNAs (see above) were ligated with one to several non-spin-labelled RNA fragments. These unlabelled RNA fragments were generated from an RNA precursor, which was obtained by in vitro transcription as previously described [27] , [28] . The RNA precursor was then subjected to sequence-specific RNase E cleavage assisted with a 2′- O -methyl-RNA/DNA chimera hybridized to the site of cleavage [27] , [28] . All the spin-labelled ( Supplementary Fig. 3 ) and non-spin-labelled RNA fragments were ligated with T4 DNA ligase using a long DNA splint covering almost the entire RNA sequence. To prevent low ligation efficiencies, the spin label should not be attached to nucleotides closer than 4 nts from the site of ligation, although ligation efficiencies close to 20% were obtained for a 4-piece ligation in which one spin label was attached only 3 nts away from one ligation site. The ligation reaction conditions were identical or similar as described previously [27] , [28] , except that the ligation reactions were performed in the absence of dithiothreitol (DTT) in the ligation buffer to prevent reduction of the spin label. Noteworthy, the ligation efficiency (typically 20–40%) was not diminished by omitting DTT. The reactions were directly loaded onto an anion-exchange HPLC followed by n -butanol extraction and lyophilization [27] , [28] . The harsh HPLC purification of the spin-labelled RNA did not lead to cleavage of the spin label. The spin-labelling efficiencies were determined by continuous wave (CW) EPR and were for most RNAs in the range 85–100%. An overview of the 4-thiouridine-modified RNAs used to obtain all the doubly spin-labelled RNAs is presented in Supplementary Fig. 3 . Preparation of protein–RNA complexes The model systems (two singly spin-labelled RNAs bound to one RsmE protein dimer) for DEER measurements were prepared by titrating a concentrated RNA solution (typically 50 μM) into concentrated protein solution (typically 1 mM) with an amount of salts such that the concentration in 30 μl results in 30 mM NaCl, 50 mM potassium phosphate at pH 7.2. After lyophilization, the complex was resuspended into 15 μl D 2 O and 15 μl deuterated glycerol to obtain 100 μM doubly spin-labelled complex. RsmZ(1–72)/RsmE 1:3 complex samples for DEER measurements were prepared by mixing a 25-μM doubly spin-labelled RsmZ(1–72) RNA dissolved in water with 3.5 equivalents of deuterated RsmE protein dimer and an amount of salts such that the concentration in 30 μl volume results in 30 mM NaCl, 50 mM potassium phosphate at pH 7.2 and 100 μM in doubly spin-labelled RNA in complex. The samples were lyophilized and re-dissolved into 15 μl D 2 O and 15 μl deuterated glycerol. Before EPR measurements, the protein–RNA complex was incubated at 37 °C and the formation of the RsmZ(1–72)/RsmE 1:3 complex was validated with a native RNA polyacrylamide gel. EPR spectroscopy RNA spin-labelling efficiencies were measured with CW EPR at X-band frequencies (9.3–9.4 GHz) using a Bruker ElexSys E500 spectrometer equipped with a Bruker super high Q resonator ER4122SHQ. The samples were placed into thin glass capillaries (~0.4 mm inner diameter, BLAUBRAND micropipettes) and EPR spectra were recorded with 100 kHz field modulation, 25 dB attenuation (200 mW full incident microwave power at 0 dB attenuation), 0.10 mT modulation amplitude, 10.24 ms time constant and 40.96 ms conversion time. The spin concentrations were calculated by recording room temperature CW EPR spectra, double integrating and comparing with the corresponding data of a reference nitroxide solution of 300 μM concentration. By comparison of spin concentration data with the optically detected RNA concentrations, spin-labelling efficiencies in the range 85–100% were computed for all single stem-loop cases and for most spin-labelled full RNAs. Nitroxide–nitroxide distances were measured using the four-pulse DEER experiment [44] (for the complexes of RsmE bound to two singly labelled RNAs and for labelling sites A, C, D, E, G—at X-band; for labelling sites B, F, H—at Q-band; for the full RNA complex distances FB, BD and AG—at Q-band). The X-band DEER measurements were performed using a Bruker Elexsys E580 X-band spectrometer with an ER4118X-MS3 resonator (microwave frequency 9.2–9.6 GHz, sample diameter 3 mm). The Q-band DEER traces were measured using a home-built spectrometer [45] with a rectangular cavity for oversized samples [46] , [47] (microwave frequency 34–36 GHz, sample diameter 3 mm). DEER measurement temperature of 50 K was set with a He-flow cryostat (ER 4118 CF, Oxford Instruments). To increase the transverse relaxation times of nitroxide spin labels, RNA complexes were prepared with partially deuterated RsmE protein. This allowed for the measurement of X-band DEER traces of a length of 8–10 μs with good signal-to-noise ratios (see Supplementary Figs 1 and 2 ). At Q-band, virtually noiseless DEER traces could be measured with a minor end artefact due to weak pulse bandwidth overlap between the pump and the observer pulses. The lengths of the DEER traces for FB, BD and AG were 12, 7 and 20 μs, respectively. In the DEER experiments at Q-band, all pulses were set to a duration of 12 ns, while at X-band the pump pulse of 12 ns and all detection pulses of 32 ns were used [47] . The first inter-pulse delay time in the DEER sequence was set to 400 ns in all cases. The second delay time (between the primary echo and the refocusing pulse) was set to a value of 7–10 μs to provide sufficient range for background correction. Typical measurement time was 20–40 h for X-band measurements and 10 h for Q-band measurements. The offset between pump and detection frequencies was +65 MHz at X-band and −85 MHz at Q-band. Fitting of DEER data and extracting distance distributions were performed with DeerAnalysis software [48] . To avoid the end artefacts mentioned above, the range for the background fit was cut at least 100 ns before the end of the DEER trace. All traces were fitted with the unrestricted distance distribution model. In each case, Tikhonov regularization [49] , [50] has been performed. The best-fit background dimensionality for all samples, except for the one with the spin label at site F, was 3±0.3, which is consistent with the uniform distribution of protein–RNA complexes in solution. For the sample F, a clearly curved background was detected, and a best-fit background dimension of 3.88 was obtained. This indicates somewhat inhomogeneous distributions of spin-labelled protein–RNA complexes with respect to each other in this sample, possibly due to a weak tendency to aggregate. Modelling spin-label distributions with CYANA Modelling the spin-label distributions of two singly spin-labelled RNAs bound to one RsmE protein dimer using CYANA was based on the solution structure of RsmE bound to two 20-mer RNA stem-loops from the hcnA mRNA [26] . In the 20-mer SL RNA, the nucleotides N and X of the ANGGAX loop motif correspond to a cytosine (C9) and a uridine (U13) residue, respectively. Two separate structure calculations were performed, one for each spin-label attachment site N or X of the common A(N)GGAX motif. The same NOE, torsion angle and hydrogen bond restraints were used as in the 20-mer RNA SL complex structure ( Fig. 1b,c and simulation 1 in Supplementary Table 1 ). For the two structure calculations, either nucleotides N (C9) or X (U13) were replaced by a 4-thiouridine linked to a IA-proxyl spin label (called URAP residue, see below). Because in the 20-mer SL RNA complex, NOEs were observed only to the H5 and H6 and not to the amine or imino protons of the C9 or U13 bases, respectively [26] , the same NOEs that were used for the C9 or U13 could be included also for the 4-thiouridine moiety replacing either C9 or U13, respectively. No restraints were included for the IA-proxyl spin label. Utilizing the same NOEs for the spin-labelled thiouridine residue and thus, assuming that the structure of the 4-thiouridinebase attached to the IA-proxyl is similar as the structure of the C9 or U13 bases in the 20-mer SL RNA complex can be rationalized by the following facts: first, the solution structures of the 20-mer RNA stem-loop bound to RsmE [26] and of five A(N)GGAX motifs present in the RsmZ RNA form Pseudomonas fluorescens CHA0 bound to RsmE [20] , show that the nucleotides N and X are not specifically recognized by the protein and indicate that the position of the base of the nucleotides N or X is similar, independent of the identity of the latter. Second, the good agreement between measured and modelled spin-label distributions ( Fig. 1 ) supports the assumption of a similar structure of the base in 4-thiouridine linked to IA-proxyl or the natural C9 or U13 bases in the 20-mer SL RNA complex. For spin-label position N or X, a structure calculation consisting of 5,000 structures and 20,000 annealing steps was performed and the 50 lowest energy structures were selected for evaluation. Using a home-written Matlab script, we determined the modelled distance distributions by plotting all 2,500 possible distances between each radical position (centre of the N–O bond in the nitroxide) in RNA 1 and RNA 2 bound to the RsmE protein and compared the modelled distance distributions with the measured DEER data. To account for the increased flexibility of nucleotide X of the common A(N)GGAX motif, we performed an additional simulation by increasing the upper limit restraints for all the intermolecular NOEs involving the thiouridine residue at nucleotide X by 2.0 Å ( Fig. 1d and simulation 2 in Supplementary Table 1 ). Because the complex of the spin-labelled RNA at position E consists of a more flexible single-stranded RNA rather than a stem-loop RNA (which is the case for all the other singly spin-labelled RNAs), we also increased for the complex spin labelled at position E the upper limits of the intra RNA NOEs involving the thiouridine residue by 2.0 Å ( Fig. 1d and simulation 3 in Supplementary Table 1 ). Construction of CYANA library for URAP residue We constructed a CYANA library for the 4-thiouridine residue to which the 3-(2-Iodoacetamido)-2,2,5,5-tetramethyl-1-pyrrolidinyloxy spin label is attached (URAP residue). First, we generated in Chem3D a standard uridine residue and the 3-(2-Iodoacetamido)-2,2,5,5-tetramethyl-1-pyrrolidinyloxy spin label. Then, both structures were connected to generate a uridine residue to which the spin label is covalently attached. Finally, we performed a MM2 minimization using Chem3D. The CYANA library for the URAP residue is presented in Supplementary Table 3 . Fixing dummy atoms into the centres of the ‘radical clouds’ For simplicity we defined the dummy atom as the CA of a glycine residue (any other protein or RNA residue could have been used), which we specified as separate molecule during structure calculation with CYANA. For each spin-label position in the full RNA in complex we defined another glycine CA dummy atom ( Fig. 3 , step 5). These dummy atoms were fixed to the geometrical centres of the ‘radical clouds’ ( Fig. 3 , step 4) by including tight lower and upper limit distance constraints between the CA of the dummy atom and several CA’s of the protein backbone of the protein dimer to which the spin-labelled RNA containing the dummy atom is bound to (see Supplementary Table 2 for a typical constraint file). Although the ‘radical cloud’ describes the spin-label conformations of a spin label attached to the RNA, we fixed the dummy atom with respect to the protein. Fixing the dummy atom with respect to the RNA might lead to distortion of the RNA structure because the RNA has a less dense net of constraints than a protein. Alternatively, the local structure of the RNA could have been fixed artificially during structure calculation such that the structure does not get distorted. Using such an approach, the dummy atom could also have been fixed with respect to the RNA. Note that not only the distance between the mean modelled and experimental distance distributions are in good agreement ( Fig. 1 ), but also the experimental mean distance is in good agreement with the distance between two dummy atoms placed into the geometrical centres of the simulated distance distributions of the model systems consisting of two singly spin-labelled RNAs bound to one RsmE protein homodimer ( Supplementary Table 1 ). This further supports the approach of constraining the geometrical centres of the spin-label distributions (described by dummy atoms) with the experimental mean distances. Cross-validation analysis We performed a cross-validation analysis to assess the importance of a certain EPR distance constraint on the outcome of the structure calculation. For each conformer L and R (see ref. 15 ) we did 21 structure calculations omitting a single distance constraint at a time. For both conformers R and L, most distance constraints could be individually omitted without significantly influencing the structural ensemble. The following distance constraints are influencing the outcome of the structure calculation: for conformer R and conformer L, omitting distance constraints BD and BE, and CF, DE, DH and GH, respectively, resulted in the generation of additional solutions. However, these additional solutions are not in agreement with the omitted distance constraint at all, supporting the fact that we found all the possible solutions that can satisfy all 21 constraints. While this analysis shows that the measurement of 21 distance constraints was sufficient to obtain a unique solution that best satisfies all 21 distance constraints and for which the measured and modelled distance distributions are in best agreement, it should be noted that it is crucial to measure a number of distance distributions large enough to prevent the risk of either missing a correct solution or obtaining more than one solution that satisfies equally well all constraints. How to cite this article: Duss, O. et al . EPR-aided approach for solution structure determination of large RNAs or protein–RNA complexes. Nat. Commun. 5:3669 doi: 10.1038/ncomms4669 (2014).